Vasculopathy-associated hyperangiotensinemia mobilizes haematopoietic stem cells/progenitors through endothelial AT2R and cytoskeletal dysregulation Patients with organ failure of vascular origin have increased circulating haematopoietic stem cells and progenitors (HSC/P). Plasma levels of angiotensin II (Ang-II), are commonly increased in vasculopathies. Hyperangiotensinemia results in activation of a very distinct Ang-II receptor set, Rho family GTPase members, and actin in bone marrow endothelial cells (BMEC) and HSC/P, which results in decreased membrane integrin activation in both BMEC and HSC/P, and in HSC/P de-adhesion and mobilization. The Ang-II effect can be reversed pharmacologically and genetically by inhibiting Ang-II production or signalling through BMEC AT 2 R, HSCP Ang-II receptor type 1 (AT 1 R)/AT 2 R or HSC/P RhoA, but not by interfering with other vascular tone mediators. Hyperangiotensinemia and high counts of circulating HSC/P seen in sickle cell disease (SCD) as a result of vascular damage, is significantly decreased by Ang-II inhibitors. Our data define for the first time the role of Ang-II HSC/P traffic regulation and redefine the haematopoietic consequences of anti-angiotensin therapy in SCD. Haematopoietic stem cells and progenitor (HSC/P) are needed constantly to replace mature blood cells. The bone marrow (BM) microenvironment regulates a homoeostatic dynamic equilibrium with a pool of circulating HSC/P [1] , [2] , [3] , [4] , [5] . The size of the circulating pool of HSC/P is critically regulated by their adhesion or de-adhesion to their microenvironment. Patients with organ failure of vasculo-endothelial origin have an increased circulating pool of HSC/P [6] , [7] , [8] and which may represent a homoeostatic stress response contributing to vascular damage repair [9] . An example of systemic vasculo-endothelial disease is sickle cell disease (SCD) which is associated with endothelial activation and damage [10] and an increased pool of circulating primitive haematopoietic progenitors [11] . Angiotensin II (Ang-II) is the major bioactive peptide of the renin–angiotensin system and is implicated in the homoeostatic regulation of blood volume, vascular tone and sodium retention [12] . Patients with vascular disease commonly develop secondary hyperangiotensinemia and BM dysfunction of multifactorial origin [13] . There is evidence for the effect of Ang-II in haematopoiesis. Studies have shown that animals and patients receiving Ang-II targeted therapies had decreased stress erythropoiesis [14] , [15] , [16] , [17] , [18] , suggesting the existence of a local Ang-II regulatory system in the BM that is involved in the regulation of haematopoiesis [19] . However, the intrinsic or extrinsic nature of the mechanisms by which Ang-II regulates HSC/P activity in pathological conditions remains unknown. In this study, we reveal that acute and chronic hyperangiotensinemia in mice results in an increased pool of circulatory HSC/P, which can be reversed pharmacologically or genetically by a microenvironmental deficiency of Ang-II receptor type 2 (AT 2 R). Hyperangiotensinemia results in HSC/P de-adhesion from BM endothelial cells (BMEC) through distinct changes in the balance of the activated Rho family GTPases, Rho and Rac, and in cytoskeletal rearrangements in the BMEC and HSC/P. We show that untreated patients with SCD have high levels of Ang-II and HSC/P in their peripheral blood, which significantly decreases on angiotensin-targeted pharmacological or genetic intervention. These results indicate a new role for angiotensin in HSC/P trafficking under pathological conditions, and define the haematopoietic consequences of anti-antigiotensin therapy in SCD. Hyperangiotensinemia increases the pool of circulating HSC/P To understand whether hyperangiotensinemia results in increased mobilization of HSC/P, we first used a murine model of chronic hyperangiotensinemia secondary to a vasculopathy. An EC deficiency of Cx43 , a gap junction forming protein that is crucial in maintaining EC-to-EC junctions and preserving the barrier function of EC, has been shown to result in chronic effective hypovolemia, hypotension and secondary hyperreninemic hyperangiotensinemia [20] . We have generated independently endothelial Cx43 -deficient mice by crossing Tie2-Cre expressing mice with biallelic Cx43 exon 2 floxed mice, demonstrated that these mice lack expression of Cx43 in BMEC, and recombined the Cx43 gene in colonies derived from peripheral blood (PB) while still expressing Cx43 in the BM stromal cells ( Supplementary Fig. 1a,b ). We have named these mice HyperAng-II ΔCx43-EC mice to summarize this dual property of deletion of Cx43 in EC and hyperangiotensinemia. HyperAng-II ΔCx43-EC mice had normal numbers of PB leucocyte subpopulations ( Supplementary Fig. 1c–f ), blood haemoglobin, and erythrocyte and platelet counts ( Supplementary Fig. 1g–i ), but had a two to threefold increase in the number of circulating myeloid committed haematopoietic progenitors ( Fig. 1a ) and repopulating stem cells ( Fig. 1b ) compared with their wild type (WT) control littermates. Immunophenotypic enumeration of circulating HSC/P in HyperAng-II ΔCx43-EC mice indicated that both the HSC and different populations of committed progenitors, including long-term HSC, short-term HSC, multipotential progenitors, common myeloid progenitors, granulo-macrophagic progenitors and megakaryoblastic-erythroid progenitors, were consistently increased two to threefold ( Supplementary Fig. 2a–e ). The increase in circulating HSC/P accounts for ~0.1% competitive repopulating units (CRU) and ~0.5% colony forming units (CFU)-C, respectively, of all BM HSC/P. These levels are similar to the mobilization with the CXCR4 inhibitor, AMD3100 (ref. 21 ). As expected, the BM content of immunophenotypically defined HSC/P ( Supplementary Fig. 2f–g ) as well as functional progenitors ( Fig. 1c ) and competitive repopulating stem cells ( Fig. 1d ) were not significantly different in HyperAng-II ΔCx43-EC mice compared with their WT control littermates, which explains the apparent absence of changes in the content of HSC/P in the BM. Similar to BM, there was no significant change in the splenic content of HSC/P in the HyperAng-II ΔCx43-EC mice ( Fig. 1e ). Interestingly, the deficiency of Cx43 in HSC/P alone does not induce HSC/P mobilization [22] , [23] , suggesting the existence of a non-cell-autonomous effect of Cx43 deficiency in HyperAng-II ΔCx43-EC mice. Generation of chimeric animals with normal haematopoiesis and Tie2-Cre;Cx43-deficient microenvironment ( Fig. 1f ) phenocopied the increased level of circulating HSC/P, confirming that the increase in circulating HSC/P in HyperAng-II ΔCx43-EC mice was of non-cell-autonomous origin ( Fig. 1g ). The increased number of circulating HSC/P in these mice was not associated with increased circulating levels of the chemokines Cxcl12 ( Supplementary Fig. 2h ) or stem cell factor ( Supplementary Fig. 2i ), which are expressed by BMEC and BM stromal cells, and are reported to function as major regulators of HSC/P content and trafficking [2] , [3] . β-adrenergic stimulation has also been shown to be critical in controlling HSC/P egress [24] . We did not observe any significant changes in the levels of norepinephrine or epinephrine in the BM ( Supplementary Fig. 2j–k ) or blood ( Supplementary Fig. 2l–m ) of HyperAng-II ΔCx43-EC mice, nor did the β-adrenergic blocker propranolol have an effect on their circulating HSC/P counts ( Supplementary Fig. 2n ). To demonstrate whether the increased level of Ang-II was responsible for the increased circulation of HSC/P, HyperAng-II ΔCx43-EC mice were given the angiotensin-converting-enzyme (ACE) inhibitor enalapril, which blocks the transformation of Ang-I into Ang-II. Enalapril was effective in reducing the plasma levels of Ang-II in HyperAng-II ΔCx43-EC mice and restored the increased count of circulating/mobilized HSC/P to levels similar to control animals ( Fig. 1h–i ), indicating that the ACE-mediated formation of Ang-II is implicated in the mobilization of HSC/P to the PB. 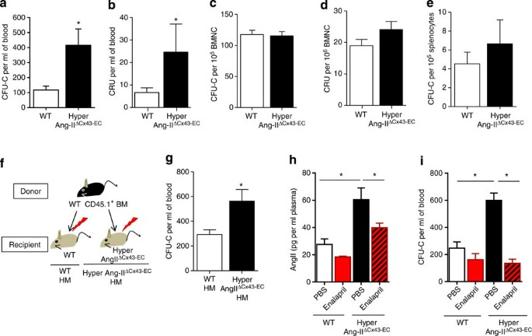Figure 1: Circulating HSC/P count is increased in chronic hyperangiotensinemia mouse model. (a) Frequency of haematopoietic progenitors in basal conditions of WT (n=10) or HyperAng-IIΔCx43-EC(n=10) mice. *P<0.05. (b) Competitive repopulating unit frequency (CRU) of stem cells in PB from WT (n=9) or HyperAng-IIΔCx43-EC(n=14) mice. *P<0.05. (c) BM CFU-C content in basal conditions of WT (n=4) or HyperAng-IIΔCx43-ECmice (n=4). (d) Frequency of BM CRU from WT (n=16) or HyperAng-IIΔCx43-ECmice (n=17) mice. (e) CFU-C in spleen from basal WT (n=3) or HyperAng-IIΔCx43-EC(n=3) mice. (f) Schema of generation of HM chimeras by transplantation of WT BM cells into WT or HyperAng-IIΔCx43-ECmice. (g) Frequency of haematopoietic progenitors in basal conditions of WT HM (n=6) or HyperAng-IIΔCx43-ECHM mice (n=6) mice. Open bars depict data from WT mice. Solid bars depict data from HyperAng-IIΔCx43-ECmice. (h) Ang-II concentration in plasma and (i) count of PB CFU-C in WT and HyperAng-IIΔCx43-ECmice treated with PBS (open bars; WT, black bars; HyperAng-IIΔCx43-EC) or enalapril (red bars; WT, hatched red bars; HyperAng-IIΔCx43-EC). Values represent mean±s.e.m. of three independent experiments, with a minimum of three mice per group and experiment. *P<0.05, Student’st-test for experiments that compare two groups or analysis of variance test with Bonferroni correction for experiments with more than two groups. Figure 1: Circulating HSC/P count is increased in chronic hyperangiotensinemia mouse model. ( a ) Frequency of haematopoietic progenitors in basal conditions of WT ( n =10) or HyperAng-II ΔCx43-EC ( n =10) mice. * P <0.05. ( b ) Competitive repopulating unit frequency (CRU) of stem cells in PB from WT ( n =9) or HyperAng-II ΔCx43-EC ( n =14) mice. * P <0.05. ( c ) BM CFU-C content in basal conditions of WT ( n =4) or HyperAng-II ΔCx43-EC mice ( n =4). ( d ) Frequency of BM CRU from WT ( n =16) or HyperAng-II ΔCx43-EC mice ( n =17) mice. ( e ) CFU-C in spleen from basal WT ( n =3) or HyperAng-II ΔCx43-EC ( n =3) mice. ( f ) Schema of generation of HM chimeras by transplantation of WT BM cells into WT or HyperAng-II ΔCx43-EC mice. ( g ) Frequency of haematopoietic progenitors in basal conditions of WT HM ( n =6) or HyperAng-II ΔCx43-EC HM mice ( n =6) mice. Open bars depict data from WT mice. Solid bars depict data from HyperAng-II ΔCx43-EC mice. ( h ) Ang-II concentration in plasma and ( i ) count of PB CFU-C in WT and HyperAng-II ΔCx43-EC mice treated with PBS (open bars; WT, black bars; HyperAng-II ΔCx43-EC ) or enalapril (red bars; WT, hatched red bars; HyperAng-II ΔCx43-EC ). Values represent mean±s.e.m. of three independent experiments, with a minimum of three mice per group and experiment. * P <0.05, Student’s t -test for experiments that compare two groups or analysis of variance test with Bonferroni correction for experiments with more than two groups. Full size image Ang-II induces HSC/P mobilization We then analyzed whether the HSC/P mobilization required chronic exposure to high levels of Ang-II or whether it could be achieved by transient hyperangiotensinemia as a result of a bolus administration of Ang-II. WT mice were administered with 1.44 mg kg −1 Ang-II dissolved in isotonic phosphate buffered saline (PBS) intraperitoneally, which resulted in increased plasma levels of Ang-II at 1, 5 and 15 min after administration, returning to basal levels by 30 min after infusion ( Supplementary Fig. 2o ). The administration of Ang-II resulted in significantly increased circulation of HSC/P in PB within 15 min post-infusion, which returned to basal levels by 30 min post-infusion ( Fig. 2a ). Furthermore, continuous infusion of Ang-II, reaching an approximately three fold increase of plasma Ang-II levels over the endogenous production ( Supplementary Fig. 2p ), resulted in concomitant increased counts of circulating HSC/P ( Fig. 2b and Supplementary Fig. 2p ). Together, this data indicated the existence of a temporal relationship between the administration of Ang-II and HSC/P mobilization to the PB of normal mice. 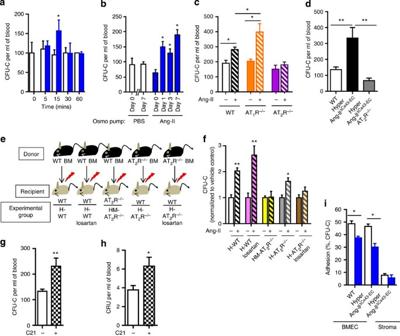Figure 2: Ang-II induces HSC/P de-adhesion and mobilization through AT2R signalling. (a) Ang-II time kinetics of HSC/P mobilization. CFU-C of Ang-II-injected mice (blue) were compared with vehicle control-treated mice (open bars) at each time point. (b) PB CFU-C counts in mice submitted to continuous infusion of Ang-II for up to 7 days. (c) WT (black outlined bars),AT1R−/−(orange bars) andAT2R−/−(purple bars) primary mice were injected with PBS (−, solid bars) or Ang-II (+, hatched bars).n=4 for each group. (d) CFU-C count in PB from WT, HyperAng-IIΔCx43-ECand AT2R-deficient-HyperAng-IIΔCx43-ECmice. (e) Schema of transplantation to generate AT2R-deficient H or HM mice. (f) Chimeric mice (H-WT, empty bars; H-WT pretreated with losartan, pink bars;HM-AT2R−/−, yellow bars;H-AT2R−/−, grey bars;H-AT2R−/−pretreated with losartan, brown bars) were injected with PBS (−, solid bars) or Ang-II (+, hatched bars). The CFU-C counts were normalized to vehicle control (−, PBS). (g,h) Circulating CFU-C and CRU in PB from mice administered vehicle control (−, PBS, open bar) or C21 (4 mg kg−1, mosaic bar). (g) CFU-C counts. Values represent mean±s.e.m. of three independent experiments with a minimum of 12 mice per group. (h) CRU counts;n=7 mice per group. (i) Adhesion of WT haematopoietic progenitors to EC from WT or HyperAng-IIΔCx43-ECmice. BM stromal cells from HyperAng-IIΔCx43-ECmice were used as a negative control. EC or stromal cells were treated with 100 μM Ang-II and the percentage of adhesion (blue bars) was compared with the adhesion of vehicle-treated cells (open bars). *P<0.05; **P<0.01, Student’st-test for experiments that compare two groups or analysis of variance test with Bonferroni correction for experiments with more than two groups. Figure 2: Ang-II induces HSC/P de-adhesion and mobilization through AT 2 R signalling. ( a ) Ang-II time kinetics of HSC/P mobilization. CFU-C of Ang-II-injected mice (blue) were compared with vehicle control-treated mice (open bars) at each time point. ( b ) PB CFU-C counts in mice submitted to continuous infusion of Ang-II for up to 7 days. ( c ) WT (black outlined bars), AT 1 R −/− (orange bars) and AT 2 R −/− (purple bars) primary mice were injected with PBS (−, solid bars) or Ang-II (+, hatched bars). n =4 for each group. ( d ) CFU-C count in PB from WT, HyperAng-II ΔCx43-EC and AT 2 R-deficient-HyperAng-II ΔCx43-EC mice. ( e ) Schema of transplantation to generate AT 2 R-deficient H or HM mice. ( f ) Chimeric mice (H-WT, empty bars; H-WT pretreated with losartan, pink bars; HM-AT 2 R −/− , yellow bars; H-AT 2 R −/− , grey bars; H-AT 2 R −/− pretreated with losartan, brown bars) were injected with PBS (−, solid bars) or Ang-II (+, hatched bars). The CFU-C counts were normalized to vehicle control (−, PBS). ( g , h ) Circulating CFU-C and CRU in PB from mice administered vehicle control (−, PBS, open bar) or C21 (4 mg kg −1 , mosaic bar). ( g ) CFU-C counts. Values represent mean±s.e.m. of three independent experiments with a minimum of 12 mice per group. ( h ) CRU counts; n =7 mice per group. ( i ) Adhesion of WT haematopoietic progenitors to EC from WT or HyperAng-II ΔCx43-EC mice. BM stromal cells from HyperAng-II ΔCx43-EC mice were used as a negative control. EC or stromal cells were treated with 100 μM Ang-II and the percentage of adhesion (blue bars) was compared with the adhesion of vehicle-treated cells (open bars). * P <0.05; ** P <0.01, Student’s t -test for experiments that compare two groups or analysis of variance test with Bonferroni correction for experiments with more than two groups. Full size image To discern whether the effect of hyperangiotensinemia is associated with its vasopressor effects, we performed experiments where we combined the infusion of Ang-II with pharmacological doses of hydralazine, a vasorelaxant with activity independent of Ang-II signalling [25] . When used at doses demonstrated to reduce blood pressure in mice (1–5 mg kg −1 ) [26] and able to counteract the vasopressor effects of Ang-II [27] , the hydralazine pre-treatment did not significantly affect the plasma levels of exogenous Ang-II ( Supplementary Fig. 3a ), and the vasorelaxant effect of 1 mg kg −1 hydralazine did not reverse the HSC/P mobilizing effect of Ang-II ( Supplementary Fig. 3b ), suggesting that the vasoconstriction effect of Ang-II was not responsible for the effect on HSC/P mobilization. This data, along with the rapid in vivo effect of the exogenous administration of Ang-II, suggest a direct effect of the hormone on Ang-II receptors. Ang-II acts through distinct ATR in different cell types Two distinct Ang-II receptor subtypes, AT 1 R and AT 2 R, which have been identified on the basis of their differential pharmacological and biochemical properties induce specific signalling pathways and seem to play distinct and sometimes opposite roles in vascular regulation [28] . Both AT 1 R and AT 2 R are expressed by BMEC and HSC/P ( Supplementary Fig. 3c ). To elucidate whether AT 1 R or AT 2 R were specifically responsible for the HSC/P mobilization phenotype, we evaluated the level of HSC/P mobilization after Ang-II administration in models of loss-of-function of Ang-II receptors. AT 1 R −/− and AT 2 R −/− mice were given a single dose of Ang-II and the level of circulating HSC/P was analyzed. While the deficiency of AT 1 R did not modify the effect of Ang-II on HSC/P mobilization, the single deficiency of AT 2 R completely prevented the increased HSC/P mobilization response after pharmacological administration of Ang-II ( Fig. 2c ), or in our model of chronic hyperangiotensinemia with AT 2 R deficiency ( Fig. 2d ), indicating that AT 2 R is indispensable to mediate the mobilization of HSC/P induced by Ang-II. To examine whether Ang-II/AT 2 R activity was cell autonomous or not, and whether the expression of other murine AT 1 R subtypes [29] may have been overlooked in our genetic murine model of AT 1 R deficiency, we generated chimeric animals by transplanting BM HSC/P from CD45.2 + WT and CD45.2 + AT 2 R −/− mice into myeloablated B6.SJL Ptprca Pepcb/BoyJ CD45.1 + recipient mice (WT and H-AT 2 R −/− , respectively). Conversely, we also generated the chimeric mice with transplantation of BM HSC/P from congenic WT CD45.1 + mice into CD45.2 + AT 2 R −/− mice (haematopoetic microenvironment (HM) HM-AT 2 R −/− ). At 6 weeks post-transplantation, fully chimeric mice (as assessed by flow cytometry) were analyzed for the effect of the genetic deficiency of AT 2 R in both haematopoietic and microenvironment compartments and for pharmacological inhibition of all AT 1 R forms (AT 1 Ra and AT 1 R) on the progenitor mobilizing response to Ang-II at 1 min post-administration ( Fig. 2e ). The single deficiency of AT 2 R in the HM prevented Ang-II-mediated HSC/P mobilization ( Fig. 2f ), demonstrating that a non-cell-autonomous effect suffices to induce Ang-II/AT 2 R-dependent HSC/P mobilization. The deficiency of AT 2 R expression in the haematopoiesis of chimeric animals within a WT microenvironment, or the administration of the AT 1 R inhibitor, losartan, to chimeric WT mice did not prevent Ang-II-mediated mobilization of HSC/P, demonstrating that haematopoietic AT 2 R or pharmacological blockade of all forms of AT 1 R did not reverse the HSC/P mobilizing effect of Ang-II. However, the combination of a genetic deficiency of HSC/P AT 2 R and the specific pharmacological blockade of AT 1 R with losartan in chimeric mice prevented the HSC/P mobilizing effect of Ang-II ( Fig. 2f ), indicating the presence of a haematopoietic intrinsic effect on Ang-II-dependent HSC/P mobilization, which can only be prevented by a combined blockade of both AT 1 R and AT 2 R. AT 2 R activation induces HSC/P mobilization Pharmacological administration of the AT 2 R agonist C21 (ref. 30 ), which specifically binds to and activates AT 2 R but has different pharmacokinetic and pharmacodynamic temporal activity from Ang-II [31] , phenocopied the effect of Ang-II on the mobilization of haematopoietic progenitors ( Fig. 2g and Supplementary Fig. 3d ) and HSC ( Fig. 2h and Supplementary Fig. 3e ) by 4 h after administration. Administration of C21 did not modify endogenous levels of Ang-II ( Supplementary Fig. 3f ) and its effect was prevented by a deficiency of AT 2 R ( Supplementary Fig. 3g ), indicating that C21 acted through an on-target effect. To identify whether Ang-II and the clinically used HSC/P mobilizer agent G-CSF collaborate in vivo , we treated C57Bl/6 mice with G-CSF (200 μg kg −1 per day) for 5 days followed by a single injection of the AT 2 R agonist C21, and determined their effect on the blood content of HSC/P using competitive repopulation and colony forming cell assays at 4 h after the administration of C21 on the 5th day of G-CSF administration. As shown in Supplementary Fig. 3h–i , no additive or negative effect was observed by the combination of G-CSF in either assay, which strongly suggested that G-CSF and Ang-II act through common signalling pathways. These data are in line with previous observations in mice where inhibition of Rac GTPase activity resulted in mobilization of HSC/P, but no additional effect of G-CSF on HSC/P mobilization was found [32] , [33] . Nitric oxide (NO) is not responsible for HSC/P mobilization HyperAng-II ΔCx43-EC mice have been shown to have increased plasma levels of NO (ref. 20 ) and Ang-II has been shown to induce NO release from EC [34] . NO levels also affect endothelial function [35] and HSC release from endothelial niches [36] . To determine whether the regulation of NO levels in HyperAng-II ΔCx43-EC mice is implicated in HSC/P mobilization, we first analyzed and confirmed the presence of increased activation levels of nitric endothelial oxide synthase (eNOS) in ex-vivo propagated BM CD45 − Ter119 − CD31 + CD106 + BMEC from WT and HyperAng-II ΔCx43-EC mice ( Supplementary Fig. 3j ). Then, we analyzed whether the exogenous administration of pharmacological doses of Ang-II or the NO scavenger, L-NG-nitroarginine methyl ester (L-NAME), to WT C57Bl/6 mice, resulted in changes in the levels of nitrates/nitrites and HSC/P in blood. Administration of either Ang-II or L-NAME reduced the plasma levels of nitrates/nitrites ( Supplementary Fig. 3k ) but L-NAME did not modify the circulating counts of HSC/P ( Supplementary Fig. 3l ). Similarly, the administration of the NO donor, S-nitroso-N-acetylpenicillamine (SNAP), to WT C57Bl/6 mice did not result in changes in the count of PB HSC/P ( Supplementary Fig. 3m ). Altogether, this data indicates that plasma NO levels do not mediate Ang-II-dependent HSC/P mobilization. Ang-II induces HSC/P de-adhesion from BMEC Adhesion of HSC/P to the endothelial microenvironment is a basic mechanism of retention and homing of HSC/P within the BM that fits the response-time associated with the rapid effect of the administration of Ang-II. BMEC and BM stromal cells of mesenchymal origin have been reported to tightly control BM homing and/or retention of HSC/P [3] , [37] . To understand whether the HSC/P adhesion to the endothelial microenvironment was impaired in the presence of Ang-II, we first analyzed if Ang-II modifies the adhesion of HSC/P to BMEC. When BMEC-adhered HSC/P were exposed to Ang-II at a concentration similar to the peak plasma level reached after the single-dose intraperitoneal administration, the fraction of BMEC-adherent HSC/P was significantly reduced ( Fig. 2i ). Confirming the independence of the effect of Ang-II on Cx43 expression, a comparable level of HSC/P de-adhesion was noticed when BMEC from either WT or HyperAng-II ΔCx43-EC mice were used ( Fig. 2i ). Interestingly, the adhesion of HSC/P to murine BM stromal cells was not reduced when cultures were exposed to Ang-II ( Fig. 2i ), suggesting that Ang-II has a specific effect on the adhesion of HSC/P to BMEC. Ang-II induces actin polymerization on BMEC and HSC/P Migration of HSC/P out of their tissue niches requires the disruption of cellular ligand–receptor adhesion molecules and/or the development of major destabilizing cytoskeletal rearrangements. Major molecular endothelial mediators of adhesion and HSC activity in the BM vascular niche are vascular cell adhesion molecule 1 (VCAM-1) (ref. 38 ) and E-selectin [39] , which have been shown to be regulated by Ang-II in other cell types [40] . Ang-II did not induce significant changes in the expression level of VCAM-1 ( Supplementary Fig. 3n ) or E-selectin (CD62e, Supplementary Fig. 3o ) on the membrane of BMEC followed for up to 15 min. In addition, cell adhesion is regulated by the dynamic reorganization of actin as well as the microtubule cytoskeleton. This involves cycles of net assembly and disassembly of actin filaments. Ang-II receptors are G protein-coupled receptors with signalling activity that induces cytoskeletal reorganization through cell-context-dependent activation or inhibition of members of the Rho family of small GTPases [41] , [42] . Therefore, we first analyzed F-actin polymerization on Ang-II stimulation of BMEC. Confocal microscopy analysis confirmed reduced focal adhesion and stress fibres, redistribution of cortical F-actin and significant morphological changes in BMEC after Ang-II exposure ( Supplementary Fig. 4a,b ). F-actin location redistributed from stress fibres to the subcortical region at 5 min after Ang-II treatment ( Supplementary Fig. 4b ). Pharmacological inhibition of Ang-II signalling using specific blockers against AT 1 R (losartan) or AT 2 R (PD123319) demonstrated that Ang-II–AT 2 R signalling in BMEC is responsible for BMEC cytoskeletal rearrangements involving cortical actin condensation, and shape changes that reduce BMEC width ( Fig. 3a–c ). Interestingly, the blockade of Ang-II–AT 1 R signalling enhanced changes in cell morphology, further reducing cell width, and increased cortical actin condensation ( Fig. 3a–c ), which may be due to the increased availability of Ang-II to bind AT 2 R. Reorganization of polymerized actin correlated with decreased Rac activation ( Fig. 3d ), increased Rho activation ( Fig. 3e ), and increased inactivation through phosphorylation of cofilin ( Supplementary Fig. 4c ), an actin-binding protein that depolymerizes actin filaments, and depends on Rac/PAK/LIMK1 activity. Altogether, this data indicate that Ang-II induces AT 2 R-dependent Rac inhibition and Rho activation in BMEC, which results in significant cytoskeletal rearrangements and cell contraction. 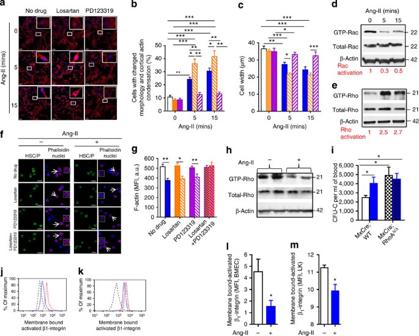Figure 3: Ang-II alters Rho GTPase family activity and expression of activated β1-integrin. (a) Representative confocal microscopic image of F-actin (phalloidin, red) and nuclear (DAPI, blue) staining of 10 μM Ang-II-treated BMEC at different time points. BMEC were pretreated with 100 nM losartan or 1 μM PD123319 or vehicle control for 1 h before Ang-II exposure. Scale bar, 50 μm. (b) Measurement of morphological changes with cortical actin condensation in BMEC with exposure of vehicle control (open, no drug treated; orange, losartan; and purple, PD123319) or Ang-II (blue, no drug; hatched orange, losartan; and hatched purple, PD123319) at different time points as shown inFig. 3a. (c) The diameter of all cells (cell width) was measured, and the average diameter of each field was calculated inFig. 3b. (d,e) Representative immunoblot of effector binding domain pull-down assay for Rac (d) or Rho A (e) in BMEC with different lengths of Ang-II exposure. (f) Representative confocal microscopic image of F-actin (phalloidin, red) and nuclear (DAPI, blue) staining of LK after 5 min exposure of 10 μM Ang-II (+). Scale bar, 10 μm. (g) The mean fluorescence intensity (MFI) of phalloidin–rhodamine in LK treated with vehicle control (solid bars) or Ang-II (hatched bars) was measured inFig. 3f. Losartan (100 nM, orange), PD123319 (1 μM, purple), combined losartan and PD123319 (orange/purple mosaic). (h) Representative immunoblot of effector binding domain pull-down assay for Rho A in LK cells with or without Ang-II treatment for 5 min. (i) CFU-C counts in PB from polyI:C-treatedMxCre; WT(solid) andRhoAflox/flox(mosaic) mice treated with Ang-II (blue) or vehicle control (PBS, black outlined). Data represent mean±s.e.m. A minimum of five mice were analyzed per group. (j,k) Representative FACS histogram of membrane-bound-activated membrane β1-integrin in BMEC (j) or LK (k) cells treated with vehicle control (red) or Ang-II (blue) and compared with isotype-treated cells (dotted line). (l,m) MFI of membrane-bound-activated membrane β1-integrin in BMEC (l) or LK (m) treated with vehicle control (open) or Ang-II (blue) was measured inFig. 2j,k. A minimum of three independent experiments were performed. *P<0.05; **P<0.01; ***P<0.001; Studentt-test for experiments that compare two groups or analysis of variance test with Bonferroni correction for experiments with more than two groups. For immunoblots, molecular weight markers in kilodalton are presented on the right side. Figure 3: Ang-II alters Rho GTPase family activity and expression of activated β1-integrin. ( a ) Representative confocal microscopic image of F-actin (phalloidin, red) and nuclear (DAPI, blue) staining of 10 μM Ang-II-treated BMEC at different time points. BMEC were pretreated with 100 nM losartan or 1 μM PD123319 or vehicle control for 1 h before Ang-II exposure. Scale bar, 50 μm. ( b ) Measurement of morphological changes with cortical actin condensation in BMEC with exposure of vehicle control (open, no drug treated; orange, losartan; and purple, PD123319) or Ang-II (blue, no drug; hatched orange, losartan; and hatched purple, PD123319) at different time points as shown in Fig. 3a . ( c ) The diameter of all cells (cell width) was measured, and the average diameter of each field was calculated in Fig. 3b . ( d , e ) Representative immunoblot of effector binding domain pull-down assay for Rac ( d ) or Rho A ( e ) in BMEC with different lengths of Ang-II exposure. ( f ) Representative confocal microscopic image of F-actin (phalloidin, red) and nuclear (DAPI, blue) staining of LK after 5 min exposure of 10 μM Ang-II (+). Scale bar, 10 μm. ( g ) The mean fluorescence intensity (MFI) of phalloidin–rhodamine in LK treated with vehicle control (solid bars) or Ang-II (hatched bars) was measured in Fig. 3f . Losartan (100 nM, orange), PD123319 (1 μM, purple), combined losartan and PD123319 (orange/purple mosaic). ( h ) Representative immunoblot of effector binding domain pull-down assay for Rho A in LK cells with or without Ang-II treatment for 5 min. ( i ) CFU-C counts in PB from polyI:C-treated MxCre; WT (solid) and RhoA flox/flox (mosaic) mice treated with Ang-II (blue) or vehicle control (PBS, black outlined). Data represent mean±s.e.m. A minimum of five mice were analyzed per group. ( j , k ) Representative FACS histogram of membrane-bound-activated membrane β1-integrin in BMEC ( j ) or LK ( k ) cells treated with vehicle control (red) or Ang-II (blue) and compared with isotype-treated cells (dotted line). ( l , m ) MFI of membrane-bound-activated membrane β1-integrin in BMEC ( l ) or LK ( m ) treated with vehicle control (open) or Ang-II (blue) was measured in Fig. 2j,k . A minimum of three independent experiments were performed. * P <0.05; ** P <0.01; *** P <0.001; Student t -test for experiments that compare two groups or analysis of variance test with Bonferroni correction for experiments with more than two groups. For immunoblots, molecular weight markers in kilodalton are presented on the right side. Full size image Ang-II differently activates Rho GTPase in BMEC and HSC/P In lung cancer-bearing mice, chronic cell-autonomous Ang-II/AT 1 R signalling has been shown to amplify the splenic content of HSC/P and macrophage progenitors [43] . To analyze the cellular mechanism of rapid HSC/P de-adhesion from BMEC, we designed co-cultures of HSC/P with WT BMEC and analyzed the level of actin polymerization in HSC/P after the addition of Ang-II. As a source of HSC/P, BM c-kit + /Sca-1 (LK) cells were used and allowed to adhere onto WT BMEC in the same manner as in Fig. 2i , and analyzed at different time points after Ang-II addition. Confocal microscopy of these co-cultures revealed reduced cortical localization of polymerized actin and an overall ~20% reduction in F-actin clustering in BM LK cells, as early as 5 min after Ang-II stimulation ( Supplementary Fig. 4d,e ), which closely preceded HSC/P de-adhesion in vitro and mobilization in vivo (as shown in Fig. 2a,i , respectively). Co-cultures of BM LK cells with BMEC demonstrated that the decrease in cortical actin polymerization of HSC/P required both AT 2 R and AT 1 R cell-autonomous signalling ( Fig. 3f,g ), suggesting that Ang-II signals through both AT 2 R and AT 1 R in HSC/P to disrupt the cytoskeletal integrity of adhered cells. Effector pull-down assays of Rho from isolated, adhered HSC/P, indicated that the activation of Rho in HSC/P was significantly decreased at 5 min after Ang-II stimulation ( Fig. 3h ), mirror imaging the Rho GTPase activation signalling of BMEC on Ang-II stimulation. Cytoskeletal and Rho activity changes were associated with activation of Rac and inhibition of myosin light chain activation ( Supplementary Fig. 4f,g ). Phenocopying the loss of RhoA induced by Ang-II, genetic deletion of HSC/P RhoA activity in an inducible murine model ( Supplementary Fig. 4h ) resulted in HSC/P mobilization at levels similar to those of HyperAng-II ΔCx43-EC mice, which was unresponsive to exogenous administration of Ang-II ( Fig. 3i ). This data strongly suggested that HSC/P Rho activity is required for Ang-II-dependent cell-autonomous HSC/P mobilization, and that the activation of HSC/P Rho signalling is dependent on both AT 1 R and AT 2 R. Ang-II reduces β1-integrin activation on the cell membrane Impaired activation of β1-integrins is dependent on a fine regulation of Rho family GTPase activity [44] and has been shown to be crucial for HSC/P adhesion to the BM microenvironment [45] . Cytoskeletal and Rho/Rac activity changes induced by Ang-II were not associated with changes in the expression or localization of membrane BMEC or HSC/P β1-integrin ( Supplementary Fig. 4i–l ) but did impair membrane β1-integrin activation in BMEC (~65% inhibition, Fig. 3j,l ) and more modestly in HSC/P (~10% inhibition, Fig. 3k,m ). Overall, this data indicates that Ang-II induces cytoskeletal dysregulation in both BMEC and HSC/P in synchronous, mirror image processes of Rho family members. Similar to other cell types [46] , [47] , the in vivo loss of Rac or Rho activity results in decreased membrane-activated membrane β1-integrin expression, resulting in HSC/P–BMEC de-coupling and de-adhesion, suggesting that this is a highly conserved mechanism of cell adhesion. Augmented HSC/P mobilization in SCD is regulated by Ang-II SCD results from substitution of a single nucleotide, valine for glutamic acid, at the sixth amino acid of the β-globin chain of haemoglobin A. SCD is characterized by globin polymerization that results in red cell dehydration, haemolysis and subsequent stress erythropoiesis. Vascular occlusions and pathology is a common feature in SCD patients [10] . There is also an increased circulatory count of primitive HSC/P in SCD patients [11] . The mechanism of endogenous mobilization of HSC/P in SCD patients has not yet been delineated, however, it has been speculated that they may be a by-product of local inflammatory responses to the underlying vasculopathy prevalent in many organ sites in SCD patients [11] . Based on the known pathobiological effects of SCD on endothelial function and our data regarding the role of Ang-II in HSC/P mobilization, we hypothesized that the increased circulation of HSC/P in SCD may be secondary to hyperangiotensinemia. To test this hypothesis, we analyzed PB specimens from SCD animals and patients. Berkeley sickle cell mice (Berk-SS) are used as animal models of human SCD, and exclusively express the human globins, human α- and β S -globin , with deletions of the murine α- and β-globin genes [48] . These mice recapitulate all the features found in humans with SCD, including irreversibly sickled red cells, anaemia and vasculopathy. Compared with WT mice (either Berk-AA or C57Bl/6 mice), Berk-SS mice had increased levels of Ang-II ( Fig. 4a ), which correlated with increased numbers of circulating HSC/P ( Fig. 4b,c and Supplementary Figs 5a–d ). A group of WT mice that had been transplanted with the BM of Berk-SS mice, also showed a significantly increased level of Ang-II compared with the WT cohorts, and when these Berk-SS/WT chimeras were administered the ACE inhibitor, captopril, the Ang-II concentrations were reduced to the level seen in WT controls ( Fig. 4d ). More interestingly, captopril-treated mice had an attenuated number of circulating HSC/P, compared with vehicle-treated Berk-SS/WT chimeric mice ( Fig. 4e ). Mechanistically, similar to our experiments in pharmacological or genetic models of hyperangiotensinemia, we analyzed whether the deficiency of microenvironment AT 2 R had any effect on the mobilization of HSC/P in Berk-SS chimeric mice. Berk-SS BM was transplanted into fully myeloablated WT or AT 2 R −/− mice to generate chimeric animals ( Supplementary Fig. 5e ). All chimeric Berk-SS mice were anaemic and showed all the haematological characteristics of primary Berk-SS mice by 6 weeks post-transplantation. Exogenous administration of Ang-II maintained its HSC/P mobilizing effect in Berk-SS/WT chimeric mice, but not in chimeric Berk-SS/AT 2 R −/− mice ( Supplementary Fig 5f ), confirming the requirement of AT 2 R expression for Ang-II-dependent mobilization in SCD mice. 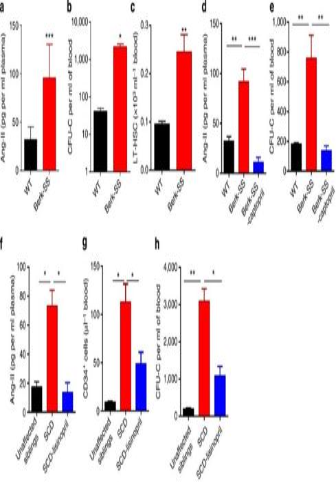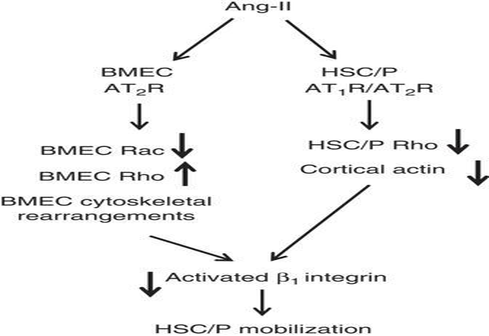Figure 5: Proposed pathway of Ang-II-induced HSC/P mobilization. On Ang-II stimulation, AT2R in EC is mainly responsible for reducing Rac activation and increasing Rho activation, resulting in increased actin polymerization and stress fibres. At the same time, cell-autonomous AT1R and AT2R downregulate Rho GTPase activity and actin polymerization in HSC/P, resulting in de-adhesion as well. Both mirror image processes of Rho GTPase activation or inhibition result in a common pathway of downregulation of the levels of activated membrane β1-integrin and consequent detachment of HSC/P from EC. Figure 4: Increased Ang-II level correlates with increased HSC/P circulation in SCD. (a) Plasma Ang-II concentration in Berkeley AA (WT, black) and Berk-SS (red) mice. ***P<0.001. Data represent mean±s.e.m. (b) CFU-C in PB from Berkeley AA (WT, black) and Berk-SS (red) mice. (c) Long-term HSC (LT-HSC) in PB from WT and Berk-SS mice. (d) Plasma Ang-II concentration in C57bl/6 mice transplanted with either the BM of AA (WT, black,n=8) or SS mice (red,n=7). Subgroup of chimeric SS mice were treated with captopril (blue,n=7). (e) CFU-C counts in PB from the mice inc. Data represent mean±s.e.m. (f) Ang-II concentration in plasma from age-matched, unaffected sibling control (black,n=8), patient with SCD (red,n=15) and SCD patient with lisinopril treatment (blue,n=4). *P<0.05. Data represent mean±s.e.m. (g) Number of circulating CD34+cells in the PB fromf. Data represent mean±s.e.m. (h) CFU-C counts in PB from (g) a healthy age-matched, unaffected sibling controls (black), patients with SCD (red) and SCD patients in treatment with lisinopril (blue). Values represent mean±s.e.m. of three independent experiments. *P<0.05. **P<0.01, ***P<0.001, Studentt-test for experiments that compare two groups, or analysis of variance test with Bonferroni correction for experiments with more than two groups. Figure 4: Increased Ang-II level correlates with increased HSC/P circulation in SCD. ( a ) Plasma Ang-II concentration in Berkeley AA (WT, black) and Berk-SS (red) mice. *** P <0.001. Data represent mean±s.e.m. ( b ) CFU-C in PB from Berkeley AA (WT, black) and Berk-SS (red) mice. ( c ) Long-term HSC (LT-HSC) in PB from WT and Berk-SS mice. ( d ) Plasma Ang-II concentration in C57bl/6 mice transplanted with either the BM of AA (WT, black, n =8) or SS mice (red, n =7). Subgroup of chimeric SS mice were treated with captopril (blue, n =7). ( e ) CFU-C counts in PB from the mice in c . Data represent mean±s.e.m. ( f ) Ang-II concentration in plasma from age-matched, unaffected sibling control (black, n =8), patient with SCD (red, n =15) and SCD patient with lisinopril treatment (blue, n =4). * P <0.05. Data represent mean±s.e.m. ( g ) Number of circulating CD34 + cells in the PB from f . Data represent mean±s.e.m. ( h ) CFU-C counts in PB from ( g ) a healthy age-matched, unaffected sibling controls (black), patients with SCD (red) and SCD patients in treatment with lisinopril (blue). Values represent mean±s.e.m. of three independent experiments. * P <0.05. ** P <0.01, *** P <0.001, Student t -test for experiments that compare two groups, or analysis of variance test with Bonferroni correction for experiments with more than two groups. Full size image To ensure that the phenomenon seen in sickle mice also occurs in humans with SCD, we analyzed the levels of Ang-II and the counts of circulating HSC/P in SCD patients and then compared them to unaffected sibling controls with both normal β-globin alleles. All plasma Ang-II levels ( Fig. 4f ), circulating numbers of CD34 + cells ( Fig. 4g ) and CFU-C in PB ( Fig. 4h ) were increased in SCD patients, and treatment with another ACE inhibitor, lisinopril, resulted in significantly decreased plasma levels of Ang-II and was associated with a corresponding 50–70% reduction in the circulating blood progenitors ( Fig. 4f–h ). Following a step-by-step approach and combining genetic and pharmacological methods, our manuscript provides a set of compelling data, demonstrating the role of high levels of plasma Ang-II in HSC/P mobilization. Mice with chronic hyperangiotensinemia secondary to vasculopathy have a two to three fold increase in the number of circulating myeloid committed haematopoietic progenitors and repopulating stem cells. The increase in circulating HSC/P accounts for ~0.1% CRU and ~0.5% CFU-C, respectively, of all BM HSC/P. These levels are similar to the mobilization with the CXCR4 inhibitor, AMD3100 (ref. 15 ). Using combinations of AT receptor knockout mice and pharmacological inhibitors, our data support a distinct role for AT 2 R in BMEC actin polymerization, which would coordinate with decreased cortical polymerized actin in HSC/P through either AT 1 R or AT 2 R. Ang-II would trigger distinct signalling pathways in HSC/P and BMEC that result in a similar outcome, which is the downregulation of activated membrane β1-integrin and HSC/P de-adhesion of HSC/P from their attachment to BMEC. The effect of Ang-II on microenvironmental cells seems to be quite specific, since Ang-II does not modify HSC/P adhesion to other cell types such as BM mesenchymal lineage cells. The translational implications of this work are self-evident. Every year, millions of patients receive anti-angiotensin therapies due to the harmful effects associated with chronic hyperangiotensinemia in cardiac, renal, or liver failure. While the ultimate fate of circulating HSC/P remains incompletely understood, there is an abundance of information on their role in innate immune regulation and tissue regeneration. Circulating HSC/P can survey peripheral organs and foster the local production of tissue-resident innate immune cells under steady-state conditions and in response to inflammatory signals [49] , [50] , [51] . An example of haematological vasculopathy is SCD, where vascular occlusions and pathology are a common feature [10] . In these patients, an increased circulatory count of primitive HSC/P is well-documented [11] in the context of sustained leukocytosis, which remains a major cause of inflammation associated morbi-mortality [10] , [52] , [53] , [54] . The absence of a relationship between NO levels and Ang-II-dependent HSC/P mobilization suggests that hyperangiotensinemia together with NO acting on HSC release from endothelial niches [36] , may act to mobilize HSC/P via different pathways that are dependent on cell context and induce divergent signalling pathways. The effects of Ang-II on cytoskeletal dysregulation of HSC/P and BMEC seem to be independently causative of HSC/P mobilization. Other possible effects of hyperangiotensinemia were found not responsible for the mobilizer effect of Ang-II. Increased vascular tone and modulation of NO levels are known effects of hyperangiotensinemia [27] , [34] . However, our data rule out the vasopressor or NO mediator effect as the mechanisms responsible for Ang-II-dependent HSC/P mobilization. β-adrenergic stimulation has also been shown to be critical at controlling HSC/P egress [24] . We did not observe any significant changes in the levels of norepinephrine or epinephrine in the BM or blood of mice with chronic hyperangiotensinemia, nor did the β-adrenergic blocker propranolol have an effect on their circulating HSC/P counts, suggesting that in the context of vasculopathy, sympathetic nervous system blockade may not counteract the effect of Ang-II. Our data indicate that hyperangiotensinemia induces HSC/P de-adhesion and mobilization through a direct effect on AT receptors in a cell-autonomous and non-cell-autonomous manner. HSC/P mobilization depends on the expression of AT 2 R in the endothelium, but not in the mesenchymal stroma of the BM microenvironment. Ang-II signals through BMEC AT 2 R, and through both AT 1 R and AT 2 R in HSC/P, resulting in distinct changes in RhoA activation and in cytoskeletal rearrangements of both BMEC and HSC/P, which results in common downregulation of the levels of active membrane β1-integrin, and HSC/P de-adhesion and mobilization ( Fig. 5 ). Gene deletion of RhoA phenocopies the mobilization effect of Ang-II, and RhoA-deficient mice become insensitive to Ang-II, suggesting that RhoA activation is indispensable for Ang-II-dependent mobilization. Figure 5: Proposed pathway of Ang-II-induced HSC/P mobilization. On Ang-II stimulation, AT 2 R in EC is mainly responsible for reducing Rac activation and increasing Rho activation, resulting in increased actin polymerization and stress fibres. At the same time, cell-autonomous AT 1 R and AT 2 R downregulate Rho GTPase activity and actin polymerization in HSC/P, resulting in de-adhesion as well. Both mirror image processes of Rho GTPase activation or inhibition result in a common pathway of downregulation of the levels of activated membrane β1-integrin and consequent detachment of HSC/P from EC. Full size image Altogether, this data indicates that hyperangiotensinemia/AT 2 R signalling plays a homoeostatic role in the control of the number of circulating progenitors in vasculopathies in general, and in SCD in particular. These studies demonstrate that acute or chronic hyperangiotensinemia results in HSC/P mobilization and represents a common pathway controlling HSC/P traffic in disease. Targeting Ang-II generation in vasculopathies and SCD may have a detrimental effect on the regenerative roles of circulating stem cells and progenitors, which, clinicians should take into account when using anti-angiotensin therapies. Animals All animals were treated in accordance with the National Institutes of Health Guide for the Care and Use of Laboratory Animals and all protocols were approved by institutional care and use committees for animal research at the Cincinnati Children’s Hospital Research Foundation. Endothelial specific- Cx43 -deficient mice were generated by crossing Tek promoter–Cre recombinase transgenic mice with biallelic Cx43 floxed mice [55] . Mx1Cre; RhoA flox/flox mice [56] were used, in which inactivation of RhoA in the whole BM as well as haematopoietic cells was induced by intraperitoneal administration of double-stranded RNA polyI:C (Amersham Pharmacia Biotech, Piscataway, NJ, USA) at a dose of 10 mg kg −1 , two doses every other day. These mice had been backcrossed for a minimum of five generations. AT 1 Ra (AT 1 R) knockout mice [57] were obtained from Jackson Laboratories, Bar Harbor, ME, USA. AT 2 R knockout mice [58] were kindly provided by Dr. Inagami (Vanderbilt University School of Medicine, Nashville, TN, USA). TekCre;Cx43 flox/flox ; AT 2 R −/− mice and their genetic littermate controls were generated by crossing TekCre;Cx43 flox/flox mice with AT 2 R knockout mice. Ubiquitin C-EGFP mice have been generated previously [59] . These mice had been backcrossed for >10 generations into C57Bl/6 mice. Berk-SS mice [48] were backcrossed for four generations into C57Bl/6 background to allow survival through adulthood. Experimental transgenic animals were male or female with ages ranging from 6 to 20 weeks. Six- to eight-week-old female WT C57Bl/6 mice were obtained commercially (Jackson Laboratory; Harlan Laboratories, Frederick, MD, USA) and used as WT donors and/or recipients of transduction-transplantation models. Human specimens PB specimens from healthy normal volunteers were obtained through Institutional Review Board-approved protocols and donor informed consents from Cincinnati Children’s Hospital Medical Center and the University of Cincinnati. PB specimens from unaffected siblings with no sickle cell trait or SCD in different phase (age ≥6 years of age) were collected through Institutional Review Board-approved protocols and donor informed consent from Cincinnati Children’s Hospital Medical Center and the University of Cincinnati. Flow cytometry analysis and sorting For the phonotypical characterization of HSC/P, low density (LD) BM cells were obtained after separation using Histopaque-1083 (Sigma, Saint Louis, MO, USA) and stained with allophycocyanin-cyanan7 (APC-Cy7)-conjugated lineage markers (CD45R (B220; clone RA3-6B2), Gr-1 (Ly-6G and Ly-6C; clone RB6-8C5), CD4 (L3T4; clone RM4-5), CD8a (Ly-2; clone 53-6.7), CD3e (clone 145-2C11), CD11b (M1/70) and Ter119 (Ly-76)), allophycocyanin (APC)-conjugated c-Kit and fluorescein isothiocyanate (FITC)-conjugated Sca-1 antibodies to identify the Lin − /c-kit + /Sca-1 + (LSK) BM cell population. IL7Rα (PE Cy7 conjugated, clone SB/199), CD34 (Pacific blue, clone RAM34), CD16/CD32 (PerCp-Cy5.5 conjugated, clone 2.4G2) and CD135 (PE conjugated, clone A2F10) were used. A sequential gating strategy on nucleated cells as discriminated by light scatter properties and sequencial gating of lineage negative LSK or LK was used. For additional subpopulations, long-term HSC were defined as LSK/CD34−/CD135−; short-term HSC were defined as LSK/CD34+/CD135− and multipotential progenitors were defined as LSK/CD34+/CD135+. For more differentiated progenitors, megakaryoblastic-erythroid progenitors were defined as LK/CD34−/CD16/CD32−; common myeloid progenitors were defined as LK/CD34+/CD16/CD32− and granulo-macrophagic progenitors were defined as LK/CD34+/CD16/CD32+ events. For sorting of BM-derived ECs, PE-conjugated CD45 and Ter119 antibodies were used along with APC-conjugated CD31 (clone MEC 13.3) and FITC-conjugated CD106 (clone 429) and sorted by flow cytometry (FACSAria II, BD Biosciences, San Jose, CA, USA). Rhodamine–phalloidin (Invitrogen), PE-conjugated β1-integrin (eBioHMb1-1) or CD62E (clone 10E9.6) and FITC-conjugated VCAM-1 (CD106, clone 429) were used and compared with isotype controls to analyze expressions of adhesion molecules in BMEC cells or sorted LK BM cells. LK or BMEC cells were treated with primary antibody against the membrane-bound active form of β1 integrin (9EG7) followed by Alexa-Fluor 647-conjugated goat anti-Rat immunoglobulin-G. The mean fluorescence intensity was normalized to that of the isotype control as a ratio. Competitive repopulation and CFU-C For the analysis of CRU in PB or BM, 200–400 μl of PB or 3 × 10 6 BM were transplanted together with 3 × 10 6 CD45.1 + BM B6.SJL Ptprca Pepcb/BoyJ (CD45.1 + ) into CD45.1 + mice. Haematopoietic cell engraftment was examined by CD45.1 and CD45.2 determination using flow cytometry analysis and analyzed at 4 months post-transplantation. Frequencies of circulating haematopoietic progenitors in PB or BM were analyzed after 9 days of methylcellulose culture (Stem Cell Technologies, Vancouver, BC, Canada). PB total and differential counts were analyzed using a Hemavet 950 (DREW Scientific, Inc., Waterbury, CT, USA). In vivo drug administration All inhibitors and antagonists were given by intraperitoneal injection. Ang-II (Sigma-Aldrich, 1.44 mg kg −1 ) and enalapril (Sigma-Aldrich, 1 mg kg −1 ) were dissolved in PBS [60] . PBS dissolved L-NAME (Sigma-Aldrich, 10 mg kg −1 ) was injected and PB was drawn at 10 min post-administration [61] . Acidic deoxygenated buffer dissolved SNAP (Cayman Chemical Co., Ann Arbor, MI, USA) was diluted in PBS (20 μg kg −1 ) and PB was collected after 20 min of injection [62] . Propranolol was dissolved in water (Sigma-Aldrich, 10 mg kg −1 ) then administrated to mice intraperitoneally and PB was collected after 20 min of injection [63] . Losartan was administered intraperitoneally (Northstar Rx LLC, Memphis, TN, USA, 50 mg kg −1 ) [64] 2 h before administration of PBS or Ang-II. Captopril (Wockhardt USA LLC, Parsippany, NJ) was mixed with drinking water (0.15 mg ml −1 for captopril) and given ad libitum in bottles that were changed twice a week. SS chimeric mice were treated with captopril for 10 weeks. Compound 21 (C21, Vicore Pharma AB, Mölndal, Sweden) was injected intraperitoneally (4 mg kg −1 ) to mice and PB was drawn post 4 h of C21 administration for analysis. G-CSF (0.2 mg kg −1 , Neupogen, Amgen Inc., Thousand Oaks, CA, USA) was daily injected intraperitoneally for 5 days. Two different doses of hydralazine (1 mg kg −1 and 5 mg kg −1 , Sigma-Aldrich) were intravenously administered with similar results and Ang-II injection was followed after 45 min post hydralazine administration [26] . For a continuous infusion of Ang-II in vivo , osmo pump (alzet mini-osmotic pump, DURECT Corporation, Cupertino, CA, USA) surgery was performed. To reach the similar plasma Ang-II concentration as one bolus of intraperitoneal injection, the pumps were filled with Ang-II (14 μg ml −1 ) or PBS as vehicle control. The osmo pumps were subcutaneously placed on the back of the mice and the mice were monitored for a week to check the plasma concentration of Ang-II and HSC/P contents in PB. HSC/P adhesion EC cells from BM of WT or HyperAng-II ΔCx43-EC mice were isolated from whole BM using FACS sorting (CD45 − /Ter119 − /CD31 + /CD106 + ) then cultured in EC growth medium-2 (EGM-2, Lonza, Walkersville, MD, USA) until freshly confluent on 24-well-plates. Stromal cells from HyperAng-II ΔCx43-EC mice were also purified and expanded as previously published by our group [22] and used in these assays. WT LDBM cells were harvested from C57Bl/6 mice and 100,000 cells were plated onto EC or stromal cells in triplicate and let to adhere for 1 h. After adhesion, co-cultures were treated with vehicle or 100 μM Ang-II for 15 min. The supernatant was removed and washed gently twice. Adhesion of BM WT HSC/P was quantified using a CFU-C assay. ELISA tests PB was collected in tubes containing EDTA and centrifuged at 3000 g for 20 min at 4 °C for immediate separation of plasma. To prevent degradation of Ang-II, an inhibitor cocktail was added and the solution was stored at −80 °C until used for the ELISA assay. Phenyl cartridge columns (ALPCO, NH) were used to extract highly purified Ang-II from the plasma. The cross-reactivity with other forms of angiotensin is comparatively low (Angiotensin I, 4%; Angiotensin 1–7, <0.001%). The concentration of Ang-II from PB was calculated according to manufacturer’s protocol (Cayman). Total nitrite and nitrate concentration were measured using freshly drawn PB from the mice, according to the manufacturer’s protocol (R&D systems, Minneapolis, MN). Soluble Cxcl12 and stem cell factor were measured in the extracellular fluid of femoral BM as previously described by our group [22] . The concentrations of norepinephrine and epinephrine in plasma as well as in femoral BM were measured according to manufacturer’s protocol (Labor Diagnostika Nord GmbH & Co. KG, Nordhorn, Germany). Western blotting and pull-down assays Lineage negative cells were purified using magnetic bead-based methods (Miltenyi Biotec, Bergisch Gladbach, Germany), and protein extracts were prepared using a radioimmunoprecipitation lysis buffer (RIPA, Cell Signaling Technology, Danvers, MA, USA), or for pull-down assays a high-Mg ++ containing buffer supplemented with protease and phosphatases inhibitor cocktails following manufacturer’s instructions (Roche Applied Science, Mannheim, Germany). GTPase activities as well as protein expression and phosphorylation were measured as previously described by our group [39] by effector binding precipitation with p21-activated kinase-bound beads (for Rac activity) and rhotekin-bound beads (for Rho activity; Cell Signaling Technology). The lysates were separated using 10% SDS–PAGE gels, transferred to polyvinylidene fluoride membranes and detected with antibodies. The primary antibodies used were: β-actin (1:6,000, clone AC-15, Sigma-Aldrich), AT 1 R (1:1,000, clone 1E10-1A9, Abcam, Cambridge, MA), AT 2 R (1:500, clone EPR3876, Abcam). Antibodies against eNOS (polyclonal, 1:1,000), phospho-eNOS (1:1,000, clone C9C3), MLC (polyclonal, 1:1,000), p-MLC (Ser19, polyclonal, 1:1,000), cofilin (1:1,000, clone D59) and p-cofillin (1:1,000, clone 77G2; Ser3) were obtained from Cell Signalling, and Cx43 (1:500, clone CX-1B1, Invitrogen), Rac (1:2,000), Rho (1:1,000) and VEGFR2 (1:500) were obtained from Millipore Corp., Billerica, MA. Gels were visualized using autoradiography and band density was analyzed (Image J software, National Institutes of Health, USA) at the expected electrophoretic moiety for each protein molecular weight. Complete, uncropped images of Western blots used for figure illustrations are provided in the Supplementary Fig. 6 . Immunofluorescence and confocal microscopy imaging The confocal images of the BMECs treated with 10 μM angiotensin for different time periods were acquired using LSM 710 (Carl Zeiss, Thornwood, NY) confocal system at × 10 optical magnification. The merged images of rhodamine–phalloidin and DAPI are presented. at 0, 5, 15 minutes Ang-II treatment, of angiotensin treatment, the cells that have morphological changes with condensation of actin filaments in the cortical region are counted, and presented as percentage of total cells in the field. At least 10 fields for each time point were counted. The diameter (width) of the cells at each time point was measured using ZEN 2010 software equipped with LSM 710 confocal system. The width of all cells in a field (Each field contains ~60–80 cells) were measured, and the average diameter of each field was calculated. For each time point, 8–10 fields of images were measured, and therefore a total of 600–800 cells were measured for the quantification of the diameter of the cells at each time point of angiotensin treatment. Bar, 50μm. Sorted LK cells stained with carboxyfluorescein succinimidyl ester (1 M, Invitrogen) or from ubiquitin C-EGFP mice were co-cultured with WT BMEC for 4 h in absence of other additives and for another an additional hour in absence or presence of 100 nM losartan, 1 μM PD123319 (Tocris Bioscience, Bristol, UK) or both. At the end of the incubation period, Ang-II was added for 5 min, before any significant HSC/P detachment occurs, and cultures were fixed with 4% formaldehyde. The stained cells were analyzed by a LSM 510 confocal system (Carl Zeiss) equipped with an inverted microscope (Observer Z1, Carl Zeiss) using a Plan Apochromat × 63, 1.4 numerical aperture oil immersion lens. Argon ion 488, HeNe 543 and HeNe633 laser lines were used to excite EGFP, rhodamine and Topro3, respectively. The acquired images were three-dimensional reconstituted, then the phalloidin–rhodamine staining on LK cells was isolated by electronically removing the phalloidin–rhodamine staining of EC (IMARIS software, Bitplane AG, Zurich, Switzerland), and were processed using Adobe Photoshop v7 (Adobe Systems Inc., San Jose, CA). Statistical analysis Quantitative data is given as mean±s.e.m. Statistical significance was determined using an unpaired Student t -test or one-way analysis of variance with Bonferroni correction. A value of P <0.05 was considered to be statistically significant. How to cite this article: Chang, K. H. et al. Vasculopathy associated hyperangiotensinemia mobilizes haematopoietic stem cells/progenitors through endothelial AT 2 R and cytoskeletal dysregulation. Nat. Commun. 6:5914 doi: 10.1038/ncomms6914 (2015).